Evidence for ligand- and solvent-induced disproportionation of uranium(IV) 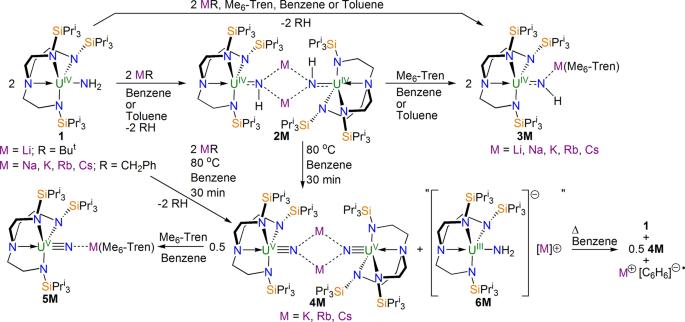Fig. 1: Synthesis of 2M–6M. Complex1is deprotonated by organo-alkali metal reagents to afford the imido dimers2M. The imido dimers2Mcan be converted to the imido monomers3Mby addition of Me6-Tren. Either isolated or in situ prepared2Mwhen heated in benzene afford the nitride dimers4M, which can be converted to the nitride monomers5Mby addition of Me6-Tren. Complexes6Mwere not isolated, but their oxidation product,1, was isolated. Disproportionation, where a chemical element converts its oxidation state to two different ones, one higher and one lower, underpins the fundamental chemistry of metal ions. The overwhelming majority of uranium disproportionations involve uranium(III) and (V), with a singular example of uranium(IV) to uranium(V/III) disproportionation known, involving a nitride to imido/triflate transformation. Here, we report a conceptually opposite disproportionation of uranium(IV)-imido complexes to uranium(V)-nitride/uranium(III)-amide mixtures. This is facilitated by benzene, but not toluene, since benzene engages in a redox reaction with the uranium(III)-amide product to give uranium(IV)-amide and reduced arene. These disproportionations occur with potassium, rubidium, and cesium counter cations, but not lithium or sodium, reflecting the stability of the corresponding alkali metal-arene by-products. This reveals an exceptional level of ligand- and solvent-control over a key thermodynamic property of uranium, and is complementary to isolobal uranium(V)-oxo disproportionations, suggesting a potentially wider prevalence possibly with broad implications for the chemistry of uranium. Disproportionation, where an ion in an oxidation state converts to ions with two different oxidation states, one higher and one lower, has fundamentally underpinned and defined the chemistry of metal ions for over two centuries [1] , [2] . Disproportionation of uranium was established 96 years ago [3] , [4] , and the status quo remained unchanged over seven decades [5] , [6] , where uranium(V) disproportionates to uranium(IV) and (VI), Eq. ( 1 ), and uranium(III) disproportionates to uranium(0) and (IV), Eq. ( 2 ). These intrinsic disproportionations, unless kinetically blocked, occur over a wide range of solvents, supporting ligands, and synthetic [7] , [8] , [9] and environmental scenarios [10] , [11] , reflecting the inherent thermodynamic instability of these two uranium oxidation states. 2 U^V (5f^1) → U^IV(5f^2)+U^VI (5f^0),(est. 1925)
 (1) 
    4 U^III (5f^3) →1 U^0 (7s^2 6d^1 5f^3)+3 U^IV(5f^2),(est. 1953)
 (2) 
    2 U^IV (5f^2) → U^III (5f^3)+U^V(5f^1), (est. 2016 and this work)
 (3) In contrast to uranium(III) and (V), uranium(IV) and (VI) are conversely regarded as the most stable oxidation states of uranium in virtually all solvent media and ligand environments [7] , [8] , [9] , [10] , [11] , [12] , [13] . Indeed, the inherent thermodynamic properties that underpin the redox processes of each oxidation state of uranium are arguably often little changed by the chemical environment defined by ligands and solvent, and they are usually at best kinetically suppressed or contained rather than being decisively materially altered. Thus, whilst uranium(III) and (V) intrinsically engage in disproportionation reactions unless kinetically blocked, disproportionation of uranium(VI) has never been demonstrated. Only as recently as 2016 was uranium(IV) discovered to be capable of disproportionating to uranium(III/V), specifically where a bridging diuranium(IV)-nitride complex reacted with methyl-triflate to give a uranium(III)-triflate and a uranium(V)-imido complex, Equation (3) [14] . However, the factors that govern that remarkable example of uranium(IV) disproportionation remain unknown. Here, we report an example of uranium(IV) disproportionation to uranium(III) and (V) (Eq. 3 ). Deprotonation of a uranium(IV)-amide to give -imido derivatives promotes, with mild heating, disproportionation to the corresponding uranium(III)-amide and uranium(V)-nitride complexes for three alkali metal salts in benzene, but not toluene, solvent. This reaction is conceptually the reverse reaction to the above example, namely imido to nitride/amide as opposed to nitride to imido/triflate. The disproportionation reaction reported here suggests an unusual level of external control over the thermodynamic properties of uranium, further diminishing the general imperviousness of uranium(IV) with respect to (III) and (V) [15] , and our results provide insight into the factors that are dictating the reactivity. The reactivity outlined here has parallels to that of uranyl(V) [10] , [11] , possibly suggesting a potentially wider prevalence in highly radiolytic and environmental scenarios [16] . Synthetic considerations We reported previously [17] that the uranium(IV)-amide complex [U IV (Tren TIPS )(NH 2 )] ( 1 , Tren TIPS = {N(CH 2 CH 2 NSiPr i 3 ) 3 } 3− ) can be deprotonated by alkali metal alkyl reagents to produce the pink uranium(IV)-imido dimers [{U IV (Tren TIPS )(μ-NH)(μ-M)} 2 ] ( 2M , M = Li, Na, K, Rb, Cs), Fig. 1 , which are insoluble in benzene or toluene at ambient conditions. However, 2M can be cleaved by addition of the capping agent N(CH 2 CH 2 NMe 2 ) 3 (Me 6 -Tren), producing the uranium(IV)-imido monomers [U IV (Tren TIPS )(μ-NH)(μ-M)(Me 6 -Tren)] ( 3M ) in crystalline yields ranging from 35 to 76%, Fig. 1 . Complexes 3M are relatively more soluble in benzene or toluene than 2M , rendering solution-state characterisation spectroscopically possible. Alternatively, 3M can be prepared from 1 in a one-pot reaction instead of separate metallation then capping steps. Throughout both these reaction sequences the oxidation state of uranium remains unchanged at +4, and these reactions all work in benzene or toluene solvents. During the course of our study, we investigated the effect of thermolysis, and found that moderate heating (80 °C) of reaction mixtures of 1 and potassium, rubidium, or caesium alkyls in benzene did not afford 2K , 2Rb , and 2Cs , respectively. Instead, a different outcome was observed, and the dark red uranium(V)-nitride dimers [{U V (Tren TIPS )(μ-N)(μ-M)} 2 ] ( 4M , M = K, Rb, Cs) [18] , [19] were isolated in crystalline yields of 18–30% (50% maximum yield for disproportionation reactions suggested by a uranium(V) product void of a N–H linkage, see below), Fig. 1 . Given their structural similarities to 2K / Rb / Cs , in order to enable meaningful comparisons to be made to monomeric 3K / Rb / Cs and further confirm the identities of 4K / Rb / Cs , we converted the latter dimeric trio to the dark red uranium(V)-nitride monomers [U V (Tren TIPS )(μ-N)(μ-M)(Me 6 -Tren)] ( 5M , M = K, Rb, Cs), and isolated them in crystalline yields of 46–76%. Fig. 1 . In contrast, treatment of 1 with lithium and sodium alkyls does not furnish 4Li and 4Na , and instead 2Li and 2Na are consistently isolated. To complete and provide a calibrated 5M series, we treated dimeric 4Li and 4Na , prepared by an established procedure [18] , with two equivalents of Me 6 -Tren to produce monomeric 5Li and 5Na . The NMR and IR spectra of 3M and 5M are consistent with their formulations (Supplementary Figs. 1–25). Fig. 1: Synthesis of 2M–6M. Complex 1 is deprotonated by organo-alkali metal reagents to afford the imido dimers 2M . The imido dimers 2M can be converted to the imido monomers 3M by addition of Me 6 -Tren. Either isolated or in situ prepared 2M when heated in benzene afford the nitride dimers 4M , which can be converted to the nitride monomers 5M by addition of Me 6 -Tren. Complexes 6M were not isolated, but their oxidation product, 1 , was isolated. Full size image Crystallographic characterisation The characterisation data and crystallographic unit cell checks for 4K / Rb / Cs produced by disproportionation match those of authentic samples [18] , [19] , [20] . The solid-state structures of the 3M and 5M series were determined, confirming their formulations, Figs. 2 and 3 (Supplementary Tables 1 – 6 ). For each complex, a triamidoamine-uranium component is bound to a central nitrogen, that resides in the pocket defined by the Tren TIPS ligand, with that nitrogen atom bridging to a Me 6 -Tren-capped alkali metal. The salient, key difference between the 3M and 5M series is the presence of a hydrogen atom on the central nitrogen of the 3M imido complexes, whereas no hydrogen atom is present in the 5M nitride series, resulting in decisively different, and characteristic, U-N imido bond lengths that average 2.007 Å (range: 1.979(4)–2.070(4) Å) for the 3M series and shorter U-N nitride distances averaging 1.810 Å (range: 1.792(4)–1.823(3) Å) for the 5M complexes. For comparison, the U-N imido distances in the 2M series span the range 2.042(3)–2.135(3) Å [17] , uranium(V)-nitride complexes of the form [U V (Tren TIPS )(μ-N)(μ-M)(crown)] exhibit U-N nitride distances spanning the range 1.803(5)–1.840(3) Å [18] , [19] , [21] , and the sum of the covalent radii for doubly and triply bonded uranium and nitrogen are 1.94 and 1.72 Å, respectively [22] . Notably, the U-N-M angles span a larger range for the 3M series (141.01(19)–175.8(2)°) compared to the 5M series (155.8(3)–177.66(18)°), consistent with the nitride ligand being a harder and less flexible ligand than imido. Fig. 2: Solid-state single crystal structures of uranium(IV)-imido (3M) complexes at 150 K with 40% probability displacement ellipsoids. a complex 3Li . b complex 3Na . c complex 3K . d complex 3Rb . e complex 3Cs . In each case all non-imido hydrogen atoms, lattice solvent molecules, and disorder components are omitted for clarity. Full size image Fig. 3: Solid-state single crystal structures of uranium(V)-nitrides (5M) at 150 K with 40% probability displacement ellipsoids. a complex 5Li . 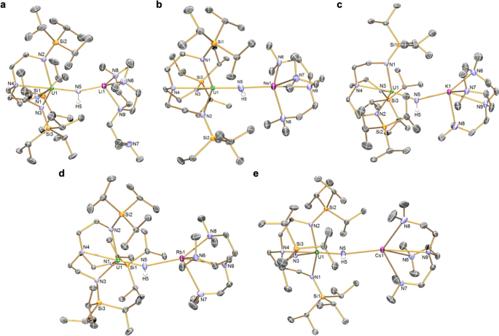Fig. 2: Solid-state single crystal structures of uranium(IV)-imido (3M) complexes at 150 K with 40% probability displacement ellipsoids. acomplex3Li.bcomplex3Na.ccomplex3K.dcomplex3Rb.ecomplex3Cs. In each case all non-imido hydrogen atoms, lattice solvent molecules, and disorder components are omitted for clarity. b complex 5Na . c complex 5K . d complex 5Rb . e complex 5Cs . 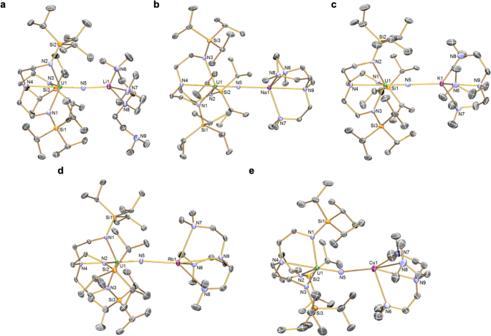Fig. 3: Solid-state single crystal structures of uranium(V)-nitrides (5M) at 150 K with 40% probability displacement ellipsoids. acomplex5Li.bcomplex5Na.ccomplex5K.dcomplex5Rb.ecomplex5Cs. In each case all non-imido hydrogen atoms, lattice solvent molecules, and disorder components are omitted for clarity. 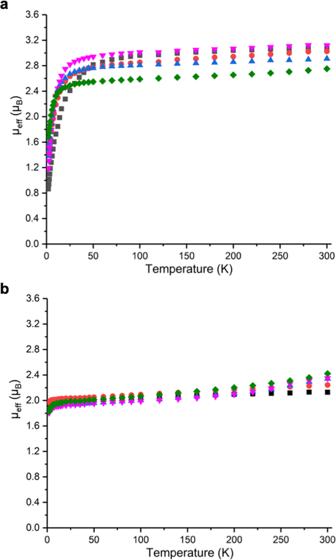Fig. 4: Variable-temperature effective magnetic moment SQUID data for uranium(IV)-imido (3M) and uranium(V)-nitride (5M) complexes. aμeff(μB) vs T (K) data in a 0.5 T external field for3Li(black squares),3Na(red circles),3K(blue triangles),3Rb(violet triangles), and3Cs(green squares).bμeff(μB) vs T (K) data in a 0.5 T external field for5Li(black squares),5Na(red circles),5K(blue triangles),5Rb(violet triangles), and5Cs(green squares). In each case all non-imido hydrogen atoms, lattice solvent molecules, and disorder components are omitted for clarity. 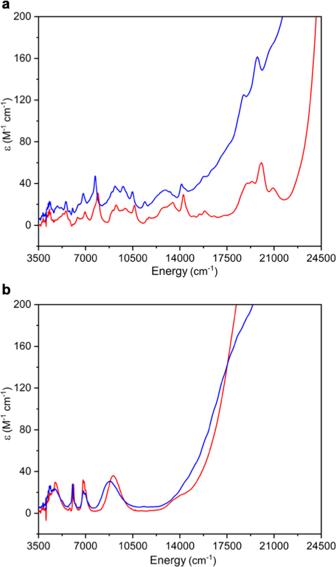Fig. 5: UV/Vis/NIR spectroscopic data for uranium(IV)-imido (3Li/Cs) and uranium(V)-nitrides (5Li/Cs) complexes. aε (M−1cm−1) vs energy (cm−1) of3Li(red trace) and3Cs(blue trace) in toluene.bε (M−1cm−1) vs energy (cm−1) of5Li(red trace) and5Cs(blue trace) in toluene. Full size image Magnetism and spectroscopic characterisation Variable-temperature superconducting quantum interference device (SQUID) magnetic and UV/Vis/NIR and NMR spectroscopic data for the 3M and 5M series confirm their formal +4 and +5 uranium oxidation states, respectively (Supplementary Figs. 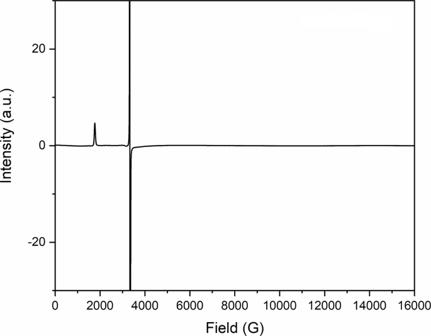Fig. 6: X-band EPR (9.44 GHz) spectrum of solid crude product from the conversion of 2K to 4K and 6K. The signal atg= 3.74 corresponds to4Kand the one atg= 2.0023 is characteristic of the benzene radical anion (linewidth 14 Gauss). 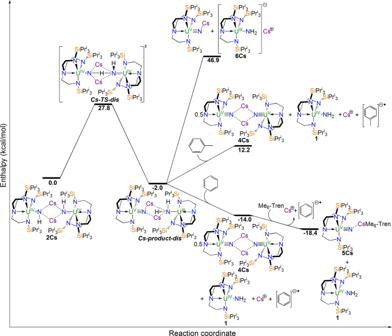Fig. 7: Computed reaction profile for the disproportionation of 2Cs to 4Cs/1/Cs+(C6H6)−•. Complex2Cscontaining two uranium(IV) ions reacts via transition stateCs-TS-disto give the disproportionation intermediateCs-product-diswhere uranium(V) and (III) ions are formed. Spontaneous cleavage ofCs-product-disto two monomer units is clearly disfavoured, as is reaction with toluene to give4Cs,1, and the caesium toluene radical anion salt.Cs-product-dishowever does react with benzene to give4Cs,1, and the caesium benzene radical anion salt. Complex4Csis then converted to5Csusing the capping agent Me6-Tren. 26–35 and Table 7 ). Specifically, the data for powdered samples of the 3M series reveal magnetic moments over the range 2.75–3.12 μ B at 300 K, Fig. 4a . These values are lower than the theoretical magnetic moment of 3.58 μ B for a 3 H 4 uranium(IV) ion [9] , [23] , but well within the range of reported magnetic moments for uranium(IV) [24] . The magnetic moments of 3M decrease little until ~50 K, then they decrease to magnetic moments spanning 0.86–1.68 μ B at 2 K. This is not classical uranium(IV) magnetism behaviour, which tends to be a smooth decrease tending to zero with a net low temperature magnetic moment of ~0.5 μ B due to temperature independent paramagnetism. However, it is characteristic of the magnetic response of uranium(IV) when bound to strong, multiply bonded donors, such as imidos [17] , carbenes [25] , [26] , phosphidos and arsenidos [27] , [28] , chalcogenidos [29] , and fluoride [30] , where the magnetic response of the 3 H 4 uranium ion, that is usually dominated by spin orbit coupling effects, is over-ridden by the ligand field [31] , [32] , [33] . In contrast, the data for powdered samples of the 5 M , Fig. 4b , series reveal magnetic moments that span 2.13–2.42 μ B at 300 K. These data are slightly reduced from the theoretical magnetic moment of 2.54 μ B for the 2 F 5/2 uranium(V) ion [9] , [23] , but are in agreement with uranium(V) magnetic moments generally [24] . The magnetic moment data for 5 M change little until ~20 K, at which point they fall sharply to magnetic moments over a narrow range of 1.81–1.97 μ B at 2 K. This behaviour is typical of classical uranium(V) where this 2 F 5/2 ion is a magnetic doublet at all temperatures, with the low temperature decrease in magnetic moment due to depopulation of low-lying paramagnetic states [9] , [23] . Fig. 4: Variable-temperature effective magnetic moment SQUID data for uranium(IV)-imido (3M) and uranium(V)-nitride (5M) complexes. a μ eff (μ B ) vs T (K) data in a 0.5 T external field for 3Li (black squares), 3Na (red circles), 3K (blue triangles), 3Rb (violet triangles), and 3Cs (green squares). b μ eff (μ B ) vs T (K) data in a 0.5 T external field for 5Li (black squares), 5Na (red circles), 5K (blue triangles), 5Rb (violet triangles), and 5Cs (green squares). Full size image The UV/Vis/NIR spectra of 3Li , 3Cs , 5Li , and 5Cs could be reliably acquired, Fig. 5 , however the others could not due to limited solubility once isolated in crystalline form. 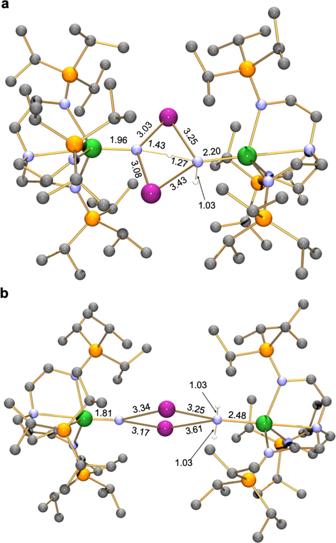Fig. 8: Computed structures, with C–H hydrogen atoms omitted for clarity, of the key transition state and intermediate in the disproportionation of 2Cs to 4Cs/1/Cs+(C6H6)−•. aThe structure ofCs-TS-diswith key bond distances (Å).bThe structure ofCs-product-diswith key bond distances (Å). Key: uranium, green; caesium, purple; carbon, grey; hydrogen, white; nitrogen, blue; silicon, orange. 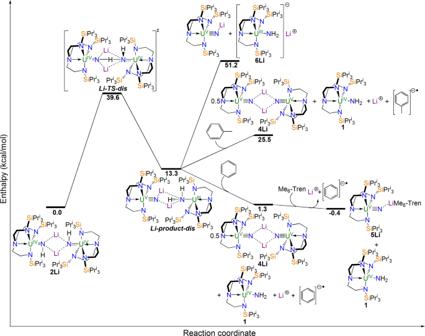Fig. 9: Computed reaction profile for the hypothetical disproportionation of 2Li to 4Li/1/Li+(C6H6)−•. Complex2Licontaining two uranium(IV) ions reacts via transition stateLi-TS-disto give the disproportionation intermediateLi-product-diswhere uranium(V) and (III) ions are formed, but this is an endothermic reaction. Spontaneous cleavage ofLi-product-disto two monomer units is clearly disfavoured, as is reaction with toluene to give4Li,1, and the lithium toluene radical anion salt. IfLi-product-disformed it would, however, react with benzene to give4Li,1, and the lithium toluene radical anion salt. Complex4Liwould then converted to5Liusing the capping agent Me6-Tren. For all complexes, strong charge transfer bands trail in from the UV region to ~17,000 cm −1 . However, for the 3Li/Cs complexes multiple and weak (ε = ≤60 M −1 cm −1 ) absorptions are present in the range 3500–17,000 cm −1 that are characteristic of intraconfigurational transitions of uranium(IV) [9] , [23] , [34] , whereas the 5Li/Cs series exhibits the fingerprint absorptions for electronic transitions between the J = 5/2 and 7/2 multiplets of the 2 F orbital manifold [35] , where J is the total angular momentum resulting from the interplay of the spin and unquenched orbital angular momenta. Where NMR data could be acquired, the 29 Si resonances of 3Li , 3Cs , 5Li , and 5Cs fall in the expected ranges for uranium(IV) and (V), respectively [36] . Fig. 5: UV/Vis/NIR spectroscopic data for uranium(IV)-imido (3Li/Cs) and uranium(V)-nitrides (5Li/Cs) complexes. a ε (M −1 cm −1 ) vs energy (cm −1 ) of 3Li (red trace) and 3Cs (blue trace) in toluene. b ε (M −1 cm −1 ) vs energy (cm −1 ) of 5Li (red trace) and 5Cs (blue trace) in toluene. Full size image Disproportionation investigation Complexes 2M and 3M are stable indefinitely in toluene or benzene at room temperature or toluene at 80 °C; only in benzene at elevated temperatures do 4K/Rb/Cs form. Complexes 4M are stable in benzene and toluene at room temperature and elevated temperatures (up to 100 °C) for days, and the eventual onset of decomposition results in the formation of Tren TIPS H 3 as the major identifiable product, but 1 is not formed. Since 4K/Rb/Cs can be obtained by heating 2K/Rb/Cs as well as in situ prepared samples, incomplete metalation of 1 and thence its presence in the reaction products can be ruled out. Thus, with the identities of 3K/Rb/Cs - 5K/Rb/Cs confirmed by the structural, spectroscopic, and magnetic characterisation data, the only plausible explanation for the formation of 4K/Rb/Cs from 1 is disproportionation of 2K/Rb/Cs and formation of the uranium(III)-amide complex [U III (Tren TIPS )(NH 2 )][M] ( 6M , M = K, Rb, Cs), which is subsequently oxidised to 1 by the benzene solvent (see below). In order to probe and confirm this aspect, we examined the disproportionation of crystalline 2K in detail. As a pink suspension of pure 2K in benzene is warmed the solution turns red as 2K dissolves, and after 30 min at 80 °C the solution becomes dark red. As the solution cools, dark red crystals of 4K grow (30% yield, 50% maximum). 1 H NMR spectroscopy reveals the presence of 1 in the mother liquor (Supplementary Fig. 36), and after work up 1 was isolated in crystalline form (38% yield, 50% maximum). When 2Rb or 2Cs are used instead of 2K , 4Rb or 4Cs along with 1 are similarly isolated. Notably, small quantities of insoluble and distinctly grey precipitates were transiently observed during reactions. The known uranium(III)-amide complex [U III (Tren TIPS )(NH 2 )][K(benzo-15-crown-5) 2 ] [37] is also distinctively grey and highly insoluble, and, notably, attempts to dissolve it in benzene by warming without exception always results in its oxidation to give solutions exclusively containing 1 , implying reduction of a sacrificial species. It is germane to note that the grey colour of [U III (Tren TIPS )(NH 2 )][K(benzo-15-crown-5) 2 ] is unique for Tren TIPS U complexes [38] , with all other derivatives being green, yellow, red, light brown, or dark blue/purple and no metal halides, that can often appear to be grey, are present in these reactions. ATR-IR spectra of crude reaction mixtures (Supplementary Fig. 37) are not inconsistent with the formation of 6K when compared to an authentic pure sample of [U III (Tren TIPS )(NH 2 )][K(benzo-15-crown-5) 2 ] [37] , but the spectra are not definitive since small variances would be expected, and do manifest, due to the crude-pure comparison. Exhaustive attempts to isolate 6K from the reaction were unsuccessful, only resulting the isolation of the oxidised product 1 . Although reaction concentrations are inherently low, immediately quenching a reaction mixture that produces 4K and 6K by freezing the benzene solution and recording an X-band (9.44 GHz) EPR spectrum reveals a weak signal at g = 2.0023 (Supplementary Fig. 38), characteristic of the benzene radical anion (linewidth 14 Gauss) [39] . Allowing the reaction to proceed longer then removing the benzene solvent and recording the X-band EPR spectrum on the solid crude product results in a spectrum with the characteristic absorption at g = 3.74 for 4 K and also a stronger signal at g = 2.0023, Fig. 6 . Replacing the benzene solvent with toluene completely blocks the production of 4K by disproportionation, and only 2K is isolated when toluene is the reaction solvent. These observations suggest that heating mixtures of 1 with heavier alkali metal alkyls promotes disproportionation of 2M to 4M and 6M (M = K, Rb, Cs). However, the latter when heated, as necessarily per the experimental conditions, spontaneously converts to 1 by reducing the benzene solvent. That this reactivity is not a viable reaction route with toluene is consistent with benzene being easier to reduce than toluene, or viewed from the opposite perspective toluene is more easily oxidised than benzene [40] . The finding that 2K , 2Rb , and 2Cs disproportionate to isolable 4K , 4Rb , and 4Cs , but 2Li and 2Na do not seem to produce 4Li or 4Na , is consistent with previous EPR spectroscopic observations that potassium, rubidium, and caesium reduce benzene, but lithium and sodium seemingly do not [39] , since the formation of the resulting lithium or sodium benzene radical anion complexes would not be favourable. Fig. 6: X-band EPR (9.44 GHz) spectrum of solid crude product from the conversion of 2K to 4K and 6K. The signal at g = 3.74 corresponds to 4K and the one at g = 2.0023 is characteristic of the benzene radical anion (linewidth 14 Gauss). Full size image Computational reaction profile analysis In order to further probe and confirm our hypothesis of uranium(IV) disproportionation to uranium(III) and (V), we modelled reaction profiles computationally at the DFT level (B3PW91) including solvent effects (Supplementary Tables 8 – 47 ). Firstly, to confirm the validity of our approach [37] , [41] , [42] , [43] , [44] , we modelled the metallation of 1 to produce 2M and 3M , for M = Li, Na, K, Cs, (Supplementary Figs. 39–42) but omitted Rb from these computationally intensive full-structure calculations since it sits in-between K and Cs. Highlighting the formation of 2Cs and 3Cs as an exemplar (Supplementary Fig. 42), deprotonation of 1 with benzyl caesium proceeds via an adduct that is 3 kcal/mol lower in energy ( Cs-adduct-in ), and negotiation of a low-lying transition state ( Cs-TS-in ) that is 3.4 kcal/mol higher in energy than Cs-adduct-in produces [U IV (Tren TIPS )(μ-NH)(Cs)] ( Cs-product-in ) that is 14.4 kcal/mol more stable than the starting point. Dimerisation to give 2Cs increases the energetic stabilisation to 25.2 kcal/mol from the starting point, and addition of Me 6 -Tren finally produces 3Cs lying 27.5 kcal/mol below the starting point, which is in-line with experimental observations. Adding further reassurance, we note in passing that the final energetic stabilities of 2M and 3M are, as expected, ordered Li > Na > K > Cs. With our reaction profile approach validated, we probed the disproportionation reactions. Again, using the Cs system as a representative example, Fig. 7 , starting with 2Cs set to zero, formation of the dinuclear, disproportionated aggregate [U V (Tren TIPS )(N)(Cs) 2 (H 2 N)(Tren TIPS )U III ] ( Cs-product-dis ), that is 2 kcal/mol lower in energy than 2Cs , is realised via a transition state ( Cs-TS-dis ) 27.8 kcal/mol above the starting point, so this intermediate is kinetically and thermodynamically accessible. Both uranium ions in Cs-TS-dis are still 5f 2 uranium(IV) (computed uranium spin densities of 2.23 and 2.18, cf 2.19 for each uranium ion in 2Cs ), and this transition state is clearly an inner-sphere hydrogen atom transfer from one imido nitrogen, an incipient nitride, to the other, a nascent amide, as revealed by inspection of the key bond metrics in Cs-TS-dis , Fig. 8 . The computed spin densities of the two uranium ions in Cs-product-dis are 1.19 and 3.12, which confirms 5f 1 and 5f 3 formulations and hence the formation of uranium(V) and (III) ions, respectively. The salient bond distances in Cs-product-dis , Fig. 8 , confirms that the nitride and amide linkages are now fully formed, which is reflected in the distinctly asymmetric Cs 2 N 2 four-membered ring of this mixed-valent complex, which contrasts to the inversion symmetric M 2 N 2 rings of homovalent 2M and 4M . The energy barrier of 27.8 kcal/mol is experimentally accessible at 80 °C, accounting for the thermally promoted nature of the disproportionation. Simple dissociation of Cs-product-dis into half an equivalent of 4Cs and 6Cs is endothermic by 48.9 kcal/mol and so is not energetically feasible nor is it experimentally observed. However, addition of benzene and its reduction by [U III (Tren TIPS )(NH 2 )][Cs] to give 4M , 1 , and the caesium salt of the benzene radical anion is energetically favourable, at 12.0 kcal/mol below the Cs-product-dis , and the formation of the benzene radical anion is experimentally observed by our EPR studies on the in-situ solution of the reaction. Further, addition of Me 6 -Tren is even more energetically stabilising by a further 4.4 kcal/mol. When benzene solvent is replaced by toluene, the production of 4M , 1 , and the caesium salt of the toluene radical anion is now disfavoured, being 14.2 kcal/mol above Cs-product-dis , which can be related to the fact that benzene is far easier to reduce than toluene; whilst this route is in principle accessible, it is ultimately an endothermic product and so does not occur. Fig. 7: Computed reaction profile for the disproportionation of 2Cs to 4Cs/1/Cs + (C 6 H 6 ) −• . Complex 2Cs containing two uranium(IV) ions reacts via transition state Cs-TS-dis to give the disproportionation intermediate Cs-product-dis where uranium(V) and (III) ions are formed. Spontaneous cleavage of Cs-product-dis to two monomer units is clearly disfavoured, as is reaction with toluene to give 4Cs , 1 , and the caesium toluene radical anion salt. Cs-product-dis however does react with benzene to give 4Cs , 1 , and the caesium benzene radical anion salt. Complex 4Cs is then converted to 5Cs using the capping agent Me 6 -Tren. Full size image Fig. 8: Computed structures, with C–H hydrogen atoms omitted for clarity, of the key transition state and intermediate in the disproportionation of 2Cs to 4Cs/1/Cs + (C 6 H 6 ) −• . a The structure of Cs-TS-dis with key bond distances (Å). b The structure of Cs-product-dis with key bond distances (Å). Key: uranium, green; caesium, purple; carbon, grey; hydrogen, white; nitrogen, blue; silicon, orange. Full size image To assess whether the experimental observations are independently reproduced computationally, we examined the conversion of 2M to 4M + 1 + M(arene) for Li, Na, and K, again omitting Rb since it sits in-between K and Cs which both give the same product outcome. We find that, with some variations of exact enthalpies, essentially the same reaction profile and outcome is computed for K (Supplementary Fig. 43) as for Cs, consistent with experiment; Rb would then evidently give the same outcome, as experimentally observed. However, when the corresponding Li and Na profiles are computed, Fig. 9 and Supplementary Information Fig. 44, we find that whilst the final, hypothetical products 5Li / Na reside at slightly lower energies than the starting points (−0.4 and −2.9 kcal/mol), the preceding 4Li / 4Na + 1 + M(arene) products are slightly positive with respect to the starting points (1.3 and 0.9 kcal/mol). As expected, for Li and Na, spontaneous cleavage of M-product-dis for Li and Na are both very unfavourable (>40 kcal/mol), underscoring the importance of the solvent in these reactions, and the toluene routes are also very unfavourable (>24 kcal/mol) compared to the starting points. All those reaction outcomes are therefore thermodynamically endothermic overall and so do not occur. Importantly, the Li-product-dis and Na-product-dis compounds are endothermic products compared to their respective starting points (13.3 and 4.5 kcal/mol) and the energy barriers are now >31 kcal/mol (cf the K and Cs congeners are <28 kcal/mol) so these intermediates are kinetically and thermodynamically disfavoured. Fig. 9: Computed reaction profile for the hypothetical disproportionation of 2Li to 4Li/1/Li + (C 6 H 6 ) −• . Complex 2Li containing two uranium(IV) ions reacts via transition state Li-TS-dis to give the disproportionation intermediate Li-product-dis where uranium(V) and (III) ions are formed, but this is an endothermic reaction. Spontaneous cleavage of Li-product-dis to two monomer units is clearly disfavoured, as is reaction with toluene to give 4Li , 1 , and the lithium toluene radical anion salt. If Li-product-dis formed it would, however, react with benzene to give 4Li , 1 , and the lithium toluene radical anion salt. Complex 4Li would then converted to 5Li using the capping agent Me 6 -Tren. Full size image The reaction profile calculations thus independently reproduce and verify the experimental hypothesis, confirming that disproportionation of uranium(IV) to uranium(III) and (V) has occurred, and that the solvent blocks or facilitates the reactivity, in the latter case also accounting for the oxidation of the uranium(III) component to uranium(IV). The regeneration of 1 from this disproportionation reaction proposed computationally also nicely independently corroborates the experimental observation that addition of an increased excess of potassium alkyl to 1 produces increased yields of 4K , because for each disproportionation event, the uranium(III) component is oxidised to 1 which under the action of further deprotonating agent in a thermolytic regime disproportionates again, generating more 4K . The reactivity disclosed here provides a complementary example of uranium(IV) disproportionation to the other example in the literature [14] . The prior report involved a diuranium(IV)-nitride complex disproportionating under the action of methyltriflate to a uranium(III)-triflate and uranium(V)-imido mixture [14] , whereas here we report a diuranium(IV)-imido disproportionating to uranium(V)-nitride and uranium(III)-amide under the action of solvent and temperature. Nitrides are typically regarded as being difficult linkages to access in the coordination sphere of actinides, so a reaction that produces a nitride, rather than a nitride reacting to give something else, is unusual. The results reported here now shed light on the factors that can induce uranium(IV) to disproportionate in as much as clearly the ligands play a key role, but the experimental and computational results both also point to the decisive role that the solvent plays in facilitating, or not, the uranium(IV) disproportionation. This constitutes an unusual level of modification of a fundamental thermodynamic property of uranium to promote a redox reaction, rather than just effecting kinetic control or blocking, in three examples by a common ligand class (imido) and widely used solvent (benzene) in combination. These external factors have shifted a fundamental redox phenomenon from unfavourable to favourable under relatively mild conditions, demonstrating a dependence on external drivers that is more reminiscent of transition metal chemistry rather than lanthanide and actinide chemistry. The establishment of two types of conceptually opposite (nitride to imido and imido to nitride) uranium(IV) disproportionation suggests the potential for elaboration, and indeed it may be a more widespread reaction pathway under more extreme conditions than is currently recognised, for example in highly radiolytic scenarios. For example, the inner-sphere proton migration during the uranium(IV) disproportionation reported here is reminiscent of proton-promoted disproportionation of di-actinyl(V) cation–cation complexes [45] , [46] , [47] , [48] , [49] , [50] that drives actinide ion mobility and complex, problematic equilibria in nuclear fuel extraction processes, e.g. PUREX [16] , and bio-mediated deposition of uranium(IV)-oxides from uranyl(VI) in the environment [10] , [11] . Tellingly, the disproportionation of uranium(IV) reported here involves H 2 N − , HN 2− , and N 3− ligands, which parallels the prevalence of isoelectronic and isolobal H 2 O, HO − , and O 2− ligands in the disproportionation chemistry of uranium(V) in cation–cation complexes [16] , [45] , so it would seem that the softer nitrogen-based ligands facilitate disproportionation with the lower oxidation state of uranium and analogously the harder oxygen-based ligands with the higher oxidation state of uranium. There are many uranium(V)-oxo complexes, including uranyl(V), and so H + -promoted disproportion of U V =O linkages is well-precedented. However, there are few U IV =NH linkages [17] , [51] , and so disproportionation of U IV =NH linkages could in principle be expanded with other ancillary ligands to Tren TIPS . Thus, the development of the third redox disproportionation reaction for uranium hints at the potential to have implications for the chemistry of uranium in a range of scientific, technological, radiochemical, and environmental scenarios. General All manipulations were carried out under an inert atmosphere of dry nitrogen using Schlenk techniques, or an MBraun UniLab glovebox operating under an atmosphere of dry nitrogen. THF, toluene and pentane solvents were dried by passage through activated alumina towers and degassed before use. Hexanes and benzene were distilled from potassium. All solvents were stored over potassium mirrors except for ethers which were stored over activated 4 Å sieves. Deuterated solvents were distilled from potassium, degassed by three freeze-pump-thaw cycles and stored under nitrogen prior to use. Bu t Li (1.0 M in pentane), and N(CH 2 CH 2 NMe 2 ) 3 were used as purchased. MCH 2 Ph (M = Na, K, Rb, Cs), [U(Tren TIPS )(NH 2 )] ( 1 ), [{U(Tren TIPS )(μ-NH)(μ-M)} 2 ] ( 2M , M = Li, Na, K, Rb, Cs), and [{U(Tren TIPS )(μ-N)(μ-M)} 2 ] ( 4M , M = Li, Na, K, Rb, Cs) were prepared using literature methods [17] , [18] , [19] , [20] , [21] , [52] . Single crystals were examined variously on either (a) an Oxford Diffraction SuperNova Atlas CCD diffractometer using mirror-monochromated MoKα radiation (λ = 0.71073 Å), (b) a Rigaku Xcalibur2 diffractometer equipped with an Atlas CCD area detector and a sealed tube source with graphite-monochromated MoKα radiation (λ = 0.71073 Å), or (c) a Rigaku FR-X diffractometer equipped with a Hypix 6HE photon counting pixel array detector with mirror-monochromated MoKα (λ = 0.71073 Å) or CuKα (λ = 1.5418 Å) radiation. Intensities were integrated from a sphere of data recorded on narrow (1.0°) frames by ω rotation. Cell parameters were refined from the observed positions of all strong reflections in each data set. Gaussian grid face-indexed absorption corrections with a beam profile correction were applied. The structures were solved either by dual methods using SHELXT [53] and all non-hydrogen atoms were refined by full-matrix least-squares on all unique F 2 values with anisotropic displacement parameters with exceptions noted in the respective cif files. Hydrogen atoms were refined with constrained geometries and riding thermal parameters; U iso (H) was set at 1.2 (1.5 for methyl groups) times U eq of the parent atom. The largest features in final difference syntheses were close to heavy atoms and were of no chemical significance. CrysAlisPro was used for control and integration [54] , and SHELXL and Olex2 were employed for structure refinement [55] , [56] . ORTEP-3 and POV-Ray were employed for molecular graphics [57] , [58] . 1 H, 29 Si{ 1 H}, and 7 Li{ 1 H} NMR spectra were recorded on a Bruker 400 spectrometer operating at 400, 79, 155 MHz, respectively; chemical shifts are quoted in ppm and are relative to TMS ( 1 H, 29 Si) and LiCl ( 7 Li). ATR-IR spectra were recorded on a Bruker Alpha spectrometer with a Platinum-ATR module in the glovebox. UV-Vis-NIR spectra were recorded on a Perkin Elmer LMD TM 750 spectrometer. Data were collected in a 1 mm path-length cuvette loaded in an MBraun glovebox and were run versus the appropriate solvent. EPR spectra were measured using a X-band (9.44 GHz) Bruker Elexsys E500 spectrometer equipped with an ER4118SMS5 resonator at 5 K. Solution samples were transferred to the quartz tubes under argon, and the tubes were flame sealed prior to experiments. Field corrections were applied to the raw data using Bruker strong pitch ( g = 2.0026) as a reference. Static variable-temperature magnetic moment data were recorded in an applied dc field of 0.5 T on by Quantum Design MPMS XL7 or MPMS 3 (for 3Li and 5Na ) SQUID magnetometers using recrystallised powdered samples. Care was taken to ensure complete thermalisation of the sample before each data point was measured and samples were immobilised in an eicosane matrix to prevent sample reorientation during measurements. Diamagnetic corrections were applied for using tabulated Pascal constants and measurements were corrected for the effect of the blank sample holders (flame sealed Wilmad NMR tube and straw) and eicosane matrix. CHN microanalyses were carried out by Martin Jennings and Anne Davies at the University of Manchester. Preparation of [U(Tren TIPS )(μ-NH)(μ-Li)(Me 6 -Tren)] (3Li) Method A: A solution of Me 6 -Tren (0.17 g, 0.75 mmol) in hexanes (5 ml) was added slowly to a pre-cooled (−78 °C) solution of Bu t Li (0.035 g, 0.55 mmol) in hexanes (10 ml). After 10 min, a solution of 1 (0.43 g, 0.50 mmol) in hexanes (10 ml) was added at −78 °C. The mixture was allowed to warm to room temperature and stirred for further 16 h, forming a red solution. All the volatiles were removed in vacuo to afford a pink solid, which was extracted in pentane (5 ml) and filtered. Pink crystals of 3Li were obtained by storing the resulting red solution at −30 °C for 2 days. Yield: 0.21 g, 38%. Method B: Me 6 -Tren (0.17 g, 0.75 mmol) was added to a pale pink suspension of 2Li (0.44 g, 0.25 mmol) in toluene (20 ml) and the reaction was stirred for 24 h at room temperature. Volatiles were removed from the resulting red solution in vacuo. The resulting solid was extracted into pentane (5 ml) and filtered; the red filtrate was stored at −30 °C for 16 h to yield pink crystals of 3Li which were isolated by decanting the mother liquor and dried in vacuo. Yield: 0.36 g, 65%. Anal. Calcd for C 45 H 106 LiN 9 Si 3 U: C, 49.02; H, 9.69; N, 11.43%. Found: C, 48.77; H, 9.99; N, 11.37%. 1 H NMR (400 MHz, C 6 D 6 , 298 K): δ −24.03 (br, 54H, CH(C H 3 ) 2 ), −23.72 (br, 9H, C H (CH 3 ) 2 ), 13.71 (br, 6H, NC H 2 CH 2 ), 18.39 (br, 18H, N(C H 3 ) 2 ), 25.04 (br, 6H, C H 2 -Me 6 -TREN), 37.50 (br, 6H, C H 2 -Me 6 -TREN), 105.44 (br, 6H, NCH 2 C H 2 ). The NH resonance was not observed in the 1 H NMR spectrum. 7 Li{ 1 H} NMR (155 MHz, 298 K, C 6 D 6 ): δ 2.03 (br). 29 Si{ 1 H} NMR (79 MHz, C 6 D 6 , 298 K): δ −155.20 (br). ATR-IR v /cm − 1 : 2935 (br, w), 2857 (m), 2823 (w), 1457 (m), 1355 (w), 1273 (w), 1115 (w), 1061 (m), 1012 (w), 931 (s), 881 (s), 733 (vs), 670 (s), 624 (m), 561 (w), 510 (w), 441 (w). The NH stretching absorption was not observed. μ eff (Evan’s method, C 6 D 6 , 298 K): 2.3 μ B . Preparation of [U(Tren TIPS )(μ-NH)(μ-Na)(Me 6 -Tren)] (3Na) Method A: A solution of Me 6 -Tren (0.17 g, 0.75 mmol) in toluene (5 ml) was added slowly to a pre-cooled (−78 °C) mixture of NaCH 2 Ph (0.063 g, 0.55 mmol) in toluene (10 ml). After 30 min, a solution of 1 (0.43 g, 0.50 mmol) in toluene (10 ml) was added at −78 °C. The mixture was allowed to warm to room temperature and stirred for further 16 h, forming a red solution. The reaction was filtered and concentrated to 5 ml. Pink crystals of 3Na were obtained by storing the resulting red solution at −30 °C for a few days. Yield: 0.26 g, 47%. Method B: Me 6 -Tren (0.17 g, 0.75 mmol) was added to a pink suspension of 2Na (0.45 g, 0.25 mmol) in toluene (20 ml) and the reaction was stirred for 24 h at room temperature. Volatiles were removed from the resulting red solution in vacuo. The resulting solid was washed with pentane (2 × 5 ml) and dried in vacuo, giving 3Na as a pink solid. Yield: 0.42 g, 76%. Anal. Calcd for C 45 H 106 NaN 9 Si 3 U: C, 48.32; H, 9.55; N, 11.27%. Found: C, 48.04; H, 9.67; N, 10.86%. 1 H NMR (400 MHz, C 6 D 6 , 298 K): δ −24.88 (br, 54H, CH(C H 3 ) 2 ), −22.56 (br, 9H, C H (CH 3 ) 2 ), 14.42 (br, 6H, NC H 2 CH 2 ), 22.29–24.13 (br, 30H, C H 2 C H 2 N(C H 3 ) 2 ), 107.21 (br, 6H, NCH 2 C H 2 ). The NH resonance was not observed in the 1 H NMR spectrum. Reliable 29 Si NMR and UV/Vis/NIR spectra and solution magnetic moment (Evan’s method) could not be obtained, due to 3Na being only partially soluble in aromatic solvent (benzene and toluene) once isolated, and it decomposes in polar solvents. ATR-IR v /cm −1 : 2936 (br, w), 2858 (m), 2825 (w), 1461 (m), 1357 (w), 1273 (w), 1116 (w), 1063 (m), 1010 (w), 934 (s), 880 (s), 735 (vs), 671 (s), 624 (m), 561 (w), 509 (w), 440 (w). The NH stretching absorption was not observed. Preparation of [U(Tren TIPS )(μ-NH)(μ-K)(Me 6 -Tren)] (3K) Method A: A solution of Me 6 -Tren (0.17 g, 0.75 mmol) in toluene (5 ml) was added slowly to a pre-cooled (−78 °C) mixture of KCH 2 Ph (0.072 g, 0.55 mmol) in toluene (10 ml). After 30 min, a solution of 1 (0.43 g, 0.50 mmol) in toluene (10 ml) was added at −78 °C. The mixture was allowed to warm to room temperature and stirred for further 16 h, forming a red solution. The mixture was filtered and concentrated to 5 ml. Pink crystals of 3K were obtained by storing the resulting red solution at −30 °C for 2 days. Yield: 0.25 g, 43%. Method B : Me 6 -Tren (0.17 g, 0.75 mmol) was added to a pink suspension of 2K (0.45 g, 0.25 mmol) in toluene (20 ml) and the reaction was stirred for 24 h at room temperature. Volatiles were removed from the resulting red solution in vacuo. The product was washed with pentane (2 × 5 ml) and dried in vacuo, giving 3K as a pink solid. Yield: 0.36 g, 63%. Anal. Calcd for C 45 H 106 KN 9 Si 3 U: C, 47.63; H, 9.42; N, 11.11%. Found: C, 47.52; H, 9.54; N, 10.65%. 1 H NMR (400 MHz, C 6 D 6 , 298 K): δ −23.74 (br, 54H, CH(C H 3 ) 2 ), −20.52 (br, 9H, C H (CH 3 ) 2 ), 15.78 (br, 6H, NC H 2 CH 2 ), 22.42 (br, 30H, C H 2 C H 2 N(C H 3 ) 2 ), 106.55 (br, 6H, NCH 2 C H 2 ). The NH resonance was not observed in the 1 H NMR spectrum. Reliable 29 Si NMR and UV/Vis/NIR spectra and solution magnetic moment (Evan’s method) could not be obtained, due to 3K being only partially soluble in aromatic solvent once isolated, and it decomposes in polar solvents. ATR-IR v /cm −1 : 2935 (br, w), 2857 (m), 2828 (w), 1460 (m), 1357 (w), 1272 (w), 1116 (w), 1066 (m), 1008 (w), 933 (s), 880 (s), 736 (vs), 670 (s), 626 (m), 558 (w), 507 (w), 442 (w). The NH stretching absorption was not observed. Preparation of [U(Tren TIPS )(μ-NH)(μ-Rb)(Me 6 -Tren)] (3Rb) Method A: A solution of Me 6 -Tren (0.17 g, 0.75 mmol) in toluene (5 ml) was added slowly to a pre-cooled (−78 °C) mixture of RbCH 2 Ph (0.097 g, 0.55 mmol) in toluene (10 ml). After 30 min, a solution of 1 (0.43 g, 0.50 mmol) in toluene (10 ml) was added at −78 °C. The mixture was allowed to warm to room temperature and stirred for further 16 h, forming a red solution. The mixture was filtered and concentrated to 5 ml. Pink crystals of 3Rb were obtained by storing the resulting red solution at −30 °C for 2 days. Yield: 0.33 g, 56%. Method B: Me 6 -Tren (0.17 g, 0.75 mmol) was added to the pink suspension of 2Rb (0.48 g, 0.25 mmol) in toluene (20 ml) and the mixture was stirred for 24 h at room temperature. Volatiles were removed from the resulting red solution in vacuo. The pink residue was washed with pentane (2 × 5 mL) and dried in vacuo, giving 3Rb as a pure pink solid. Yield: 0.40 g, 68%. Anal. Calcd for C 45 H 106 RbN 9 Si 3 U: C, 45.76; H, 9.05; N, 10.67%. Found: C, 45.71; H, 9.29; N, 10.54%. 1 H NMR (400 MHz, C 6 D 6 , 298 K): δ −23.24 (br, 54H, CH(C H 3 ) 2 ), −21.08 (br, 9H, C H (CH 3 ) 2 ), 8.54 (br, 12H, C H 2 -Me 6 -TREN), 11.03 (br, 18H, N(C H 3 ) 2 ), 16.54 (br, 6H, NC H 2 CH 2 ), 106.59 (br, 6H, NCH 2 C H 2 ). The NH resonance was not observed in the 1 H NMR spectrum. Reliable 29 Si NMR and UV/Vis/NIR spectra and solution magnetic moment (Evan’s method) could not be obtained, due to 3Rb being only partially soluble in aromatic solvent once isolated, and it decomposes in polar solvents. ATR-IR v /cm −1 : 2934 (br, w), 2880 (m), 2821 (w), 1460 (m), 1339 (w), 1274 (w), 1117 (w), 1070 (m), 1010 (w), 931 (s), 881 (s), 736 (vs), 670 (s), 624 (m), 539 (w), 508 (w), 440 (w). The NH stretching absorption was not observed. Preparation of [U(Tren TIPS )(μ-NH)(μ-Cs)(Me 6 -Tren)] (3Cs) Method A: A solution of Me 6 -Tren (0.17 g, 0.75 mmol) in toluene (5 ml) was added slowly to a pre-cooled (−78 °C) mixture of CsCH 2 Ph (0.12 g, 0.55 mmol) in toluene (10 ml). After 30 min, a solution of 1 (0.43 g, 0.50 mmol) in toluene (10 ml) was added at −78 °C. The mixture was allowed to warm up to room temperature and stirred for further 16 h, forming a dark red brown solution. The mixture was filtered and concentrated to 3 ml. Pink crystals of 3Cs were obtained by storing the resulting dark red brown solution in at −30 °C for 2 days. Yield: 0.22 g, 35%. Method B: Me 6 -Tren (0.17 g, 0.75 mmol) was added to a pink suspension of 2Cs (0.50 g, 0.25 mmol) in toluene (20 ml) and the reaction was stirred for 24 h at room temperature. Volatiles were removed from the resulting dark red brown solution in vacuo. The mixture was washed with pentane (2 × 5 mL) and dried in vacuo, giving 3Cs as a pure pink solid. Yield: 0.38 g, 60%. Anal. Calcd for C 45 H 106 CsN 9 Si 3 U: C, 43.99; H, 8.70; N, 10.26%. Found: C, 43.75; H, 8.89; N, 9.78%. 1 H NMR (400 MHz, C 6 D 6 , 298 K): δ −23.06 (br, 54H, CH(C H 3 ) 2 ), −22.03 (br, 9H, C H (CH 3 ) 2 ), 8.53 (br, 6H, C H 2 -Me 6 -TREN), 8.61 (br, 6H, C H 2 -Me 6 -TREN), 10.83 (br, 18H, N(C H 3 ) 2 ), 16.87 (br, 6H, NCH 2 C H 2 ), 108.04 (br, 6H, NCH 2 C H 2 ). The NH resonance was not observed in the 1 H NMR spectrum. 29 Si{ 1 H} NMR (79 MHz, C 6 D 6 , 298 K): δ −166.29 (br). ATR-IR v /cm −1 : 2937 (br, w), 2856 (m), 2823 (w), 1459 (m), 1357 (w), 1272 (w), 1118 (w), 1070 (m), 1010 (w), 932 (s), 880 (s), 733 (vs), 670 (s), 626 (m), 560 (w), 505 (w), 441 (w). The NH stretching absorption was not observed. μ eff (Evans method, C 6 D 6 , 298 K): 2.9 μ B . Preparation of [U(Tren TIPS )(μ-N)(μ-Li)(Me 6 -Tren)] (5Li) Me 6 -Tren (0.17 g, 0.75 mmol) was added to a red suspension of 4Li (0.44 g, 0.25 mmol) in toluene (20 ml) and the mixture was stirred for 24 h at room temperature. Volatiles were removed from the resulting red solution in vacuo. The mixture was extracted into pentane (5 ml), filtered, and the dark red filtrate was stored at −30 °C for 2 days to yield dark red crystals of 5Li , which was isolated by decanting the mother liquor and dried in vacuo. Yield: 0.38 g, 68%. Anal. Calcd for C 45 H 105 LiN 9 Si 3 U: C, 49.06; H, 9.61; N, 11.44%. Found: C, 49.13; H, 10.13; N, 11.23%. 1 H NMR (400 MHz, C 6 D 6 , 298 K): δ −26.27 (s, 9H, C H (CH 3 ) 2 ), −8.01 (s, 54H, CH(C H 3 ) 2 ), 7.50 (br, 6H, NC H 2 CH 2 ), 9.24 (br, 18H, N(C H 3 ) 2 ), 9.95 (br, 6H, C H 2 -Me 6 -TREN), 13.55 (br, 6H, C H 2 -Me 6 -TREN), 41.70 (br, 6H, NCH 2 C H 2 ). 7 Li{ 1 H} (155 MHz, 298 K, C 6 D 6 ): δ not observed. 29 Si{ 1 H} NMR (79 MHz, C 6 D 6 , 298 K): δ −15.38. FTIR v /cm −1 : 2936 (br, w), 2856 (m), 2831 (w), 1456 (m), 1354 (w), 1293 (w), 1272 (w), 1114 (w), 1058 (m), 1011 (w), 930 (s), 880 (s), 782 (w), 728 (vs), 669 (s), 625 (m), 564 (w), 510 (w), 444 (w). μ eff (Evan’s method, C 6 D 6 , 298 K): 1.6 μ B . Preparation of [U(Tren TIPS )(μ-N)(μ-Na)(Me 6 -Tren)] (5Na) Me 6 -Tren (0.17 g, 0.75 mmol) was added to a red suspension of 4Na (0.45 g, 0.25 mmol) in toluene (20 ml) and the reaction was stirred for 24 h at room temperature. Volatiles were removed from the resulting red solution in vacuo. The product was extracted into hot toluene (80 °C, 10 ml), filtered, and the dark red filtrate was stored at −30 °C for 16 h to yield dark red crystals of 5Na which was isolated by decanting the mother liquor and dried in vacuo. Yield: 0.23 g, 41%. Anal. Calcd for C 45 H 105 NaN 9 Si 3 U: C, 48.36; H, 9.47; N, 11.28%. Found: C, 48.31; H, 9.79; N, 10.51%. 1 H NMR (400 MHz, C 6 D 6 , 298 K): δ −25.05 (s, 9H, C H (CH 3 ) 2 ), −7.69 (s, 54H, CH(C H 3 ) 2 ), 7.89 (br, 6H, NC H 2 CH 2 ), 8.83 (br, 6H, C H 2 -Me 6 -TREN), 9.60 (br, 18H, N(C H 3 ) 2 ), 9.95 (br, 6H, C H 2 -Me 6 -TREN), 41.21 (br, 6H, NCH 2 C H 2 ). ATR-IR v /cm −1 : 2935 (br, w), 2857 (m), 2826 (w), 1458 (m), 1356 (w), 1300 (w), 1274 (w), 1224 (w), 1161 (w), 1116 (m), 1026 (w), 934 (s), 878 (s), 783 (w), 732 (vs), 670 (s), 627 (m), 563 (w), 510 (w), 444 (w). Reliable 29 Si NMR and UV/Vis/NIR spectra and solution magnetic moment (Evan’s method) could not be obtained as 5Na is only partially soluble in aromatic solvent once isolated, and it decomposes in polar solvents. Preparation of [U(Tren TIPS )(μ-N)(μ-K)(Me 6 -Tren)] (5K) Benzene (60 ml) was added slowly to a pre-cooled (−78 °C) mixture of 1 (0.87 g, 1.00 mmol) and KCH 2 Ph (0.13 g, 1.00 mmol). The frozen mixture was allowed to thaw to room temperature and stirred for 24 h, resulting in a pink suspension. The mixture was assayed by 1 H NMR spectroscopy, confirming that 1 was completely consumed and converted to 2K . The mixture was then heated to 80 °C for 30 min, and the mixture turned dark red. Dark red crystals of 4K started to form upon cooling the mother liquor, which was left to further crystallise at 10 °C for 16 h. The identity of 4K was confirmed by crystallographic unit cell check. Yield: 0.27 g, 30% (based on uranium). Removal of the volatiles from the mother liquor in vacuo gave a pale brown solid containing 1 as the main product by 1 H NMR spectroscopy. Pentane (2 ml) was added to the brown residue, and after filtration, a brown solution was obtained. Storing the solution at −30 °C for 24 h gave brown crystals 1 , which were isolated by filtration and dried in vacuo. Yield: 0.41 g, 47% (based on uranium). If the ratio of KCH 2 Ph is increased (by 1.5, 2.0, or even 3.0) in the first step, 4K can be isolated in higher yield (52%, based on uranium), accompanied by a lower yield of 1 (28%, based on uranium) isolated from the mother liquor. The crystalline 4K was slurried in benzene (15 ml), and Me 6 -Tren (0.10 g, 0.45 mmol) was added. The mixture was stirred for 24 h at room temperature. The red solution was concentrated to 5 ml and filtered. Slow evaporation of the red solution in a glove box afforded dark red crystals of 5K which were isolated by filtration and dried in vacuo. Yield: 0.21 g, 62%. Utilising authentic 4K produced 5K with an identical result. Anal. Calcd for C 45 H 105 KN 9 Si 3 U: C, 47.67; H, 9.34; N, 11.12%. Found: C, 47.44; H, 9.69; N, 10.92%. 1 H NMR (400 MHz, C 6 D 6 , 298 K): δ −23.81 (s, 9H, C H (CH 3 ) 2 ), −6.92 (s, 54H, CH(C H 3 ) 2 ), 6.85 (br, 30H, C H 2 C H 2 N(C H 3 ) 2 ), 8.80 (br, 6H, NCH 2 CH 2 ), 40.47 (br, 6H, NCH 2 C H 2 ). FTIR v /cm −1 : 2934 (br, w), 2855 (m), 2824 (w), 1460 (m), 1356 (w), 1310 (w), 1271 (w), 1251 (w), 1157 (w), 1068 (m), 1009 (w), 931 (s), 879 (s), 786 (w), 730 (vs), 668 (s), 626 (m), 561 (w), 507 (w), 443 (w). Reliable 29 Si NMR and UV/Vis/NIR spectra and solution magnetic moment (Evan’s method) could not be obtained as 5K is only partially soluble in aromatic solvent once isolated, and it decomposes in polar solvents. Preparation of [U(Tren TIPS )(μ-N)(μ-Rb)(Me 6 -Tren)] (5Rb) Benzene (60 ml) was added slowly to a pre-cooled (−78 °C) mixture of 1 (0.87 g, 1.00 mmol) and RbCH 2 Ph (0.18 g, 1.00 mmol). The frozen mixture was left to thaw to room temperature and stirred for 24 h, resulting in a pink suspension. The mixture was then heated to 80 °C for 30 min, and the resulting red suspension was filtered to give a dark red solution. Dark red crystals of 4Rb started to form upon cooling the mother liquor, which was left to further crystallise at 10 °C for 16 h. The identity of 4Rb was confirmed by crystallographic unit cell check. Yield: 0.22 g, 24% (based on uranium). The crystalline 4Rb was slurried in benzene (15 ml), and Me 6 -Tren (0.08 g, 0.36 mmol) was added. The mixture was stirred for 24 h at room temperature. The red solution was concentrated to 5 ml and filtered. Slow evaporation of the red solution in a glovebox afforded dark red crystals of 5Rb which were isolated by filtration and dried in vacuo. Yield: 0.22 g, 76%. Utilising authentic 4Rb produced 5Rb with an identical result. Anal. Calcd for C 45 H 105 RbN 9 Si 3 U: C, 45.80; H, 8.97; N, 10.68%. Found: C, 45.94; H, 9.30; N, 10.51%. 1 H NMR (400 MHz, C 6 D 6 , 298 K): δ −23.08 (s, 9H, C H (CH 3 ) 2 ), −6.46 (s, 54H, CH(C H 3 ) 2 ), 6.28 (br, 6H, C H 2 -Me 6 -TREN), 6.45 (br, 6H, C H 2 -Me 6 -TREN), 8.04 (br, 24H, NC H 2 CH 2 and N(C H 3 ) 2 ), 39.27 (br, 6H, NCH 2 C H 2 ). FTIR v /cm −1 : 2934 (br, w), 2855 (m), 2824 (w), 1460 (m), 1357 (w), 1301 (w), 1156 (w), 1116 (w), 1069 (m), 1009 (w), 931 (s), 879 (s), 787 (w), 731 (vs), 668 (s), 625 (m), 561 (w), 506 (w), 443 (w). Reliable 29 Si NMR and UV/Vis/NIR spectra and solution magnetic moment (Evan’s method) could not be obtained as 5Rb is only partially soluble in aromatic solvent once isolated, and it decomposes in coordinative or polar solvents. Preparation of [U(Tren TIPS )(μ-N)(μ-Cs)(Me 6 -Tren)] (5Cs) Benzene (30 ml) was added slowly to a pre-cooled (−78 °C) mixture of 1 (0.87 g, 1.00 mmol) and CsCH 2 Ph (0.34 g, 1.5 mmol). The frozen mixture was left to thaw to room temperature and stirred for 24 h, resulting in a pink suspension. The mixture was then heated to 80 °C for 30 min, and the resulting red suspension was filtered to give a red solution. Dark red crystals of 4Cs started to form upon cooling the mother liquor, which was left to further crystallise at 10 °C for 16 h. The identity of 4Cs was confirmed by crystallographic unit cell check. Yield: 0.18 g, 18% (based on uranium). The crystalline 4Cs was slurried in benzene (15 ml), and Me 6 -Tren (0.06 g, 0.27 mmol) was added. The mixture was stirred for 24 h at room temperature. Volatiles were removed from the resulting red brown solution in vacuo. The red brown residue was washed with pentane (5 ml), and then extracted into toluene (5 ml), filtered, concentrated to 2 ml, and then stored at −30 °C for 16 h to yield dark red crystals of 5Cs which were isolated by filtration and dried in vacuo. Yield: 0.10 g, 46%. Utilising authentic 4Cs produced 5Cs with an identical result. Anal. Calcd for C 45 H 105 CsN 9 Si 3 U: C, 44.03; H, 8.62; N, 10.27%. Found: C, 43.85; H, 8.92; N, 10.08%. 1 H NMR (400 MHz, C 6 D 6 , 298 K): δ −22.57 (br, d, 9H, C H (CH 3 ) 2 ), −5.98 (s, 54H, CH(C H 3 ) 2 ), 4.03 (br, 6H, C H 2 -Me 6 -TREN), 4.20 (br, 6H, C H 2 -Me 6 -TREN), 4.45 (br, 18H, N(C H 3 ) 2 ), 8.14 (br, 6H, NC H 2 CH 2 ), 37.45 (br, 6H, NCH 2 C H 2 ). 29 Si{ 1 H} NMR (79 MHz, C 6 D 6 , 298 K): δ −17.00. FTIR v /cm −1 : 2935 (br, w), 2880 (m), 2822 (w), 1460 (m), 1357 (w), 1303 (w), 1155 (w), 1118 (w), 1071 (m), 1010 (w), 930 (s), 880 (s), 786 (w), 729 (vs), 667 (m), 626 (m), 561 (w), 506 (w), 443 (w). μ eff (Evan’s method, C 6 D 6 , 298 K): 2.3 μ B . Computational details All calculations were carried out at the DFT level of theory using the hybrid functional B3PW91 [59] , [60] , with the Gaussian 09 suite of programmes [61] . The U, Th, Si and Cs atoms were represented with a small-core Stuttgart–Dresden relativistic effective core potential associated with their adapted basis set [62] , [63] , [64] . All the other atoms Li, C, H, and N were described with a 6–31 G (d,p), double-ζ quality basis set [65] , [66] , [67] , [68] . The nature of the extrema (minimum) was established with analytical frequencies calculations and geometry optimisations were computed without any symmetry constraints. The SMD solvation model was used to evaluate solvation energies by a self-consistent reaction field approach based on accurate numerical solutions of the Poisson−Boltzmann equation [69] . Benzene was chosen as solvent. The enthalpy energy was computed at T = 298 K. Intrinsic Reaction Coordinates were carried out to verify the connections of the optimised transition states.